R-Spondin 2 signalling mediates susceptibility to fatal infectious diarrhoea Citrobacter rodentium is a natural mouse pathogen widely used as a model for enteropathogenic and enterohemorrhagic Escherichia coli infections in humans. While C. rodentium causes self-limiting colitis in most inbred mouse strains, it induces fatal diarrhoea in susceptible strains. The physiological pathways as well as the genetic determinants leading to susceptibility have remained largely uncharacterized. Here we use a forward genetic approach to identify the R-spondin2 gene as a major determinant of susceptibility to C. rodentium infection. Robust induction of R-spondin2 expression during infection in susceptible mouse strains causes a potent Wnt-mediated proliferative response of colonic crypt cells, leading to the generation of an immature and poorly differentiated colonic epithelium with deficiencies in ion-transport components. Our data demonstrate a previously unknown role of R-spondins and Wnt signalling in susceptibility to infectious diarrhoea and identify R-spondin2 as a key molecular link between infection and intestinal homoeostasis. Enteropathogenic Escherichia coli (EPEC) and enterohemorrhagic Escherichia coli (EHEC) are closely related human-specific diarrhoeal pathogens that are important causes of morbidity and mortality worldwide, especially in young children [1] , [2] . EPEC and EHEC cause characteristic Attaching and Effacing (A/E) lesions in the infected intestine with tight attachment of bacteria to enterocytes, effacement of microvilli structures and profound remodelling of intestinal epithelium and mucosae [3] , [4] . Despite evidence of variability in disease severity and clinical outcome of EPEC and EHEC infections [5] , [6] , little is known about the mechanisms that regulate host susceptibility to these important pathogens. The mouse-specific pathogen C. rodentium is recognized as a good model for EPEC and EHEC [7] and can be used to study the genes implicated in host response to A/E pathogens [8] . Following C. rodentium infection, the inbred strains C3H/HeJ [8] (hereafter called C3), C3H/HeOuJ [9] (hereafter called C3Ou) and FVB [10] display high levels of mortality, while C57BL/6 (B6) mice develop self-limiting colitis [9] . Transcriptome analysis in total colonic samples from resistant or susceptible infected mice identified a common pathogenic mechanism in C3Ou and FVB mice that implicates decreased levels of expression of the major colonic HCO 3 − /Cl − exchanger Slc26a3 and the carbonic anhydrase IV ( Car4 ) together with fluid loss in faeces and perturbations in electrolyte absorption [11] . Accordingly, susceptible animals can be rescued by intensive fluid therapy [12] . We previously reported a genome-wide search carried out in cohorts of F2 progeny of susceptible C3Ou or C3 and resistant B6 mice that led to the identification of a major genetic locus on chromosome 15 controlling mortality during C. rodentium infection, which we called Cri1 (ref. 13 ). Further genotype segregation analyses in F2 (B6 x FVB) [14] populations implicate Cri1 as the common genetic cause of susceptibility of C3, C3Ou and FVB mice. Generation of congenic mice with an introgressed segment of chromosome 15 from resistant B6 genome on the susceptible C3Ou genomic background (C3Ou.B6- Cri1 ) confirmed the effect of Cri1 with full survival of congenic animals and revealed that susceptibility to C. rodentium infection was independent of the bacterial load carried by the host during disease [13] . Here, we perform genetic, physical, bioinformatic and functional dissection of the Cri1 locus and identify pathological Rspo2 -mediated Wnt activation as a major contributor to mortality following C. rodentium infection in mice. R-spondins have been implicated in intestinal morphogenesis, proliferation and carcinogenesis: our data demonstrate a previously unknown role for these proteins in the response to intestinal infection. Cri1 mediates susceptibility of AKR/J and B6.C3Ou- Cri1 mice In addition to C3, C3Ou, and FVB mice, we noted that the AKR/J strain exhibited innate susceptibility to C. rodentium infection, with a mortality rate of 66% by day 30 post infection ( Supplementary Fig. S1 ). To assess whether susceptibility of AKR/J mice was conferred by the Cri1 locus, we generated an F2 (B6 × AKR/J) population, infected with C. rodentium , and monitored survival. Mice were genotyped at rs3683812, a single-nuleotide polymorphism (SNP) marker located at the peak of Cri1 . Mice homozygous or heterozygous for AKR/J alleles at this marker suffered 63% and 58% mortality, respectively, whereas mice homozygous for B6 alleles displayed 4% mortality, clearly demonstrating a role for Cri1 in the susceptibility of AKR/J mice following C. rodentium infection ( Supplementary Fig. S2 ). Thus, Cri1 is the common genetic cause of susceptibility of the only four inbred mouse strains known to be hyper-susceptible to C. rodentium infection (C3, C3Ou, FVB and AKR). As described in the introduction, generation of congenic mice with an introgressed segment of chromosome 15 from resistant B6 genome on the susceptible C3Ou genomic background (C3Ou.B6- Cri1 ) confirmed the effect of Cri1 with full survival of congenic animals. To test the effect of Cri1 on the B6 background, we introgressed a region of chromosome 15 containing Cri1 from the susceptible C3Ou genome into the resistant B6 background (B6.C3Ou- Cri1 ). Forty-five per cent of congenic animals succumbed to infection between days 13 and 28 post infection ( Supplementary Fig. S3a,b ). Thus, despite modifying effects of the background genome, the genetic origin of Cri1 is a major determinant of C. rodentium infection outcome. Implication of Rspo2 in Cri1 -mediated susceptibility Two subcongenic lines, derived from resistant C3Ou.B6- Cri1 congenic mice and characterized by recombinations within Cri1 , were used to refine the localization of the Cri1 locus ( Fig. 1a ). Mice from the subcongenic A line (congenic region 41.20–68.76 Mb) were resistant to infection (100% survival, 30 days post infection), whereas in the subcongenic B line (congenic region 45.16–62.47 Mb), the introgression of segments from the resistant B6 genome had no effect on survival, leading to 92% mortality of this strain after 14 days of C. rodentium infection. These results unambiguously localize Cri1 to a ~4-Mb interval ( Fig. 1a ). 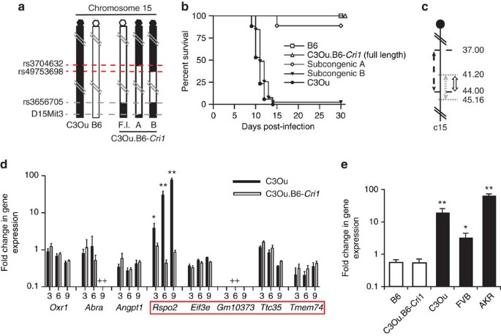Figure 1: Positional cloning of theCri1locus and identification of theRspo2gene as a major candidate gene for susceptibility toC. rodentiuminfection. (a) Genetic map of congenic and subcongenic C3Ou.B6-Cri1mice. Black indicates regions from C3Ou genome and white indicate regions from B6 genome. (b) Survival of B6, C3Ou, congenic and subcongenic C3Ou.B6-Cri1mice following oral infection withC. rodentium.C3Ou.B6-Cri1(diamonds) and subcongenic A mice (open triangles) show high levels of resistance, whereas subcongenic B mice (filled triangles) are nearly completely susceptible. These results pinpointCri1localization to an interval between marker rs3704632 and marker rs49753698 (n>15). (c) Mapping ofCri1by linkage analysis (black dotted arrow) and genetic dissection using subcongenic mice (grey dotted arrow) restrict the candidate region (white arrow). (d) Expression of all genes within the candidate region was assayed by qPCR in whole colon tissues on C3Ou and C3Ou.B6-Cri1left untreated or at indicated time after infection; results are expressed as the expression fold variation in infected mice versus untreated littermates (n≥4) at day 3, 6 and 9 post infection. ++=not detected. (e)Rspo2expression in B6, C3Ou, C3Ou.B6-Cri1, AKR and FVB mice (n=6) after 6 days of infection withC. rodentium. Data are representative of three experiments. Error bars in histograms represent s.e.m. *P<0.05; **P<0.01 (Mann–Whitney test) here and for all figures. Statistical differences between pairs of survival curves of mice grouped by genotype were calculated using log-rank test. Figure 1: Positional cloning of the Cri1 locus and identification of the Rspo2 gene as a major candidate gene for susceptibility to C. rodentium infection. ( a ) Genetic map of congenic and subcongenic C3Ou.B6- Cri1 mice. Black indicates regions from C3Ou genome and white indicate regions from B6 genome. ( b ) Survival of B6, C3Ou, congenic and subcongenic C3Ou.B6- Cri1 mice following oral infection with C. rodentium. C3Ou.B6- Cri1 (diamonds) and subcongenic A mice (open triangles) show high levels of resistance, whereas subcongenic B mice (filled triangles) are nearly completely susceptible. These results pinpoint Cri1 localization to an interval between marker rs3704632 and marker rs49753698 ( n >15). ( c ) Mapping of Cri1 by linkage analysis (black dotted arrow) and genetic dissection using subcongenic mice (grey dotted arrow) restrict the candidate region (white arrow). ( d ) Expression of all genes within the candidate region was assayed by qPCR in whole colon tissues on C3Ou and C3Ou.B6- Cri1 left untreated or at indicated time after infection; results are expressed as the expression fold variation in infected mice versus untreated littermates ( n ≥4) at day 3, 6 and 9 post infection. ++=not detected. ( e ) Rspo2 expression in B6, C3Ou, C3Ou.B6- Cri1 , AKR and FVB mice ( n =6) after 6 days of infection with C. rodentium . Data are representative of three experiments. Error bars in histograms represent s.e.m. * P <0.05; ** P <0.01 (Mann–Whitney test) here and for all figures. Statistical differences between pairs of survival curves of mice grouped by genotype were calculated using log-rank test. Full size image To identify the genetic determinant within this interval, we prioritized the region of overlap of the 95% confidence intervals defined by our previous genome-wide analyses [13] ( Fig. 1c ). Haplotype analysis of this prioritized region identified a common and specific haplotype block shared by susceptible mice and absent from resistant mouse strains that encompasses only five genes: the proximal region of Rspo2 (including the first two exons), Eif3e , Gm10373 , Ttc35 and Tmem74 ( Supplementary Fig. 4 ). We performed sequencing analyses of these five prioritized candidate genes and found no coding differences between susceptible and resistant strains. Expression of all the candidate genes was determined by qPCR in colonic samples from susceptible C3Ou mice or resistant C3Ou.B6 -Cri1 mice left uninfected or at several time points after infection ( Fig. 1d ). We found the Rspo2 gene to be rapidly, strongly and continuously induced during infection in susceptible C3Ou mice, whereas no upregulation of Rspo2 transcript was observed in resistant congenic mice. None of the other candidates were differentially regulated in C3Ou versus C3Ou.B6- Cri1 mice, nor were the genes Angpt1, Abra and Oxr1 , which are located centromeric to Rspo2 , outside of the prioritized haplotype, but still within the minimal interval delineated by genetic and physical mapping ( Fig. 1d ). We further examined Rspo2 expression during C. rodentium infection in resistant B6 mice as well as in susceptible AKR and FVB mice and found that upregulation of Rspo2 during infection is a common and specific feature of all mouse strains displaying Cri1 -mediated susceptibility to C. rodentium infection, ( Fig. 1e ) including the B6.C3Ou- Cri1 susceptible mice ( Supplementary Fig. S3c ). Rspo2 expression in colonic subepithelial stromal cells Rspo2 encodes a member of the R-Spondin family of secreted proteins (R-spondin 1–4) involved in β-catenin activation through the canonical Wnt pathway [15] . R-spondins were initially described as mitogens for epithelial cells of the mouse gastrointestinal tract [15] , [16] . Recent work has revealed an important role for R-Spondin proteins in the maintenance of intestinal stem cells in vitro via their interaction with Lgr5 receptors [17] , and transcriptionally activating gene fusions involving RSPO2 and RSPO3 have been found associated with 10% of colon tumours in humans [18] . However, the cellular source of R-Spondin and the mechanisms that regulate R-Spondin expression within the intestine remain largely uncharacterized. To investigate the cellular source of Rspo2 during C. rodentium infection, we performed reciprocal bone marrow (BM) chimera experiments with susceptible C3Ou and resistant C3Ou.B6- Cri1 congenic mice. We found that the radio-resistant (non-hematopoietic) compartment conferred both mortality following infection and Rspo2 induction in the chimeric mice ( Fig. 2a ). This is consistent with previous work [11] , suggesting that Cri1 -mediated susceptibility is not associated with disregulation of the immune response. 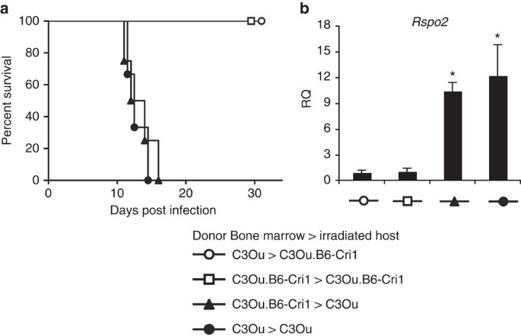Figure 2:Cri1-mediated susceptibility toC. rodentiuminfection and colonic expression ofRspo2are controlled by radio-resistant cells. (a) Survival curve of reciprocal bone marrow chimera mice infected withC. rodentiumdemonstrate that susceptibility to infection is independent of bone marrow-transferred cells but depends on the genotype of the irradiated host (n>4). (b) Relative quantification (RQ) ofRspo2expression assessed by qPCR in colonic tissues from reciprocal bone marrow chimeric mice at 7 days post infection withC. rodentium(n=4). Data represent one of two experiments. Error bars in histograms represent s.e.m. *P<0.05 (Mann-Whitney test). Figure 2: Cri1 -mediated susceptibility to C. rodentium infection and colonic expression of Rspo2 are controlled by radio-resistant cells. ( a ) Survival curve of reciprocal bone marrow chimera mice infected with C. rodentium demonstrate that susceptibility to infection is independent of bone marrow-transferred cells but depends on the genotype of the irradiated host ( n >4). ( b ) Relative quantification (RQ) of Rspo2 expression assessed by qPCR in colonic tissues from reciprocal bone marrow chimeric mice at 7 days post infection with C. rodentium ( n =4). Data represent one of two experiments. Error bars in histograms represent s.e.m. * P <0.05 (Mann-Whitney test). Full size image We next used in situ hybridization (ISH) on formalin-fixed, paraffin-embedded (FFPE) colon sections from infected C3Ou and C3Ou.B6- Cri1 mice to localize Rspo2 -expressing cells. Rspo2 expression was only readily detectable in infected susceptible C3Ou mice ( Fig. 3a ), where evident labelling of cells within the lamina propria was observed ( Fig. 3b ). Combined ISH and immunohistochemistry revealed that Rspo2 transcripts were expressed in a cell population including α-smooth muscle actin (α-SMA)- positive intestinal myofibroblasts but excluding Gr1+-infiltrating neutrophils ( Fig. 3c ). Together, these results provide evidence that during C. rodentium infection of susceptible mice, Rspo2 expression is induced in subepithelial stromal cells, but not in intestinal epithelial cells or radio-sensitive hematopoietic immune cells. 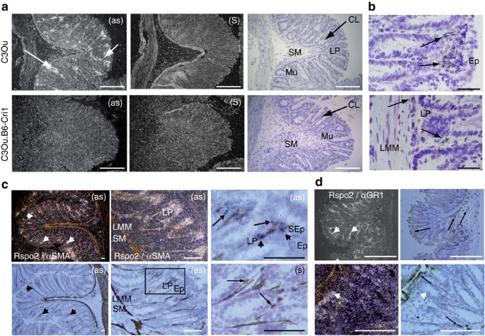Figure 3:Cri1controlsC. rodentium-inducedRspo2expression within the colonic lamina propria. (a) Emulsion autoradiography detection ofRspo2mRNA antisense labelling (as) byin situhybridization (ISH) or control (s) hybridization in the colon mucosa seen as bright under dark-field illumination in susceptible C3Ou or resistant C3Ou.B6-Cri1 at 6 days post infection. Signal was detected in the microscopical loci seen in the bottom (large arrow) and close to luminal pole (small arrow) of the lamina propria; the same sections with cresyl violet staining (right). Scale bar 200 μm. (b) Enlarged view ofRspo2-positive cells in infected susceptible C3Ou mice, ISH labelling (arrow) is observed in the lamina propria, close to the colonic epithelia (top) and at the bottom of the gland (bottom). Scale bar 50 μm. (c) Comparative localization ofRspo2mRNA and α-SMA in the colon of susceptible C3Ou mice 7 days post infection, seen at various magnification levels under dark-field (top left, top middle) or bright-field illumination (bottom left, bottom middle). Top right panel is an enlargement of the boxed area in the bottom middle panel. Bottom right panel is a control with sense labelling. Large arrowheads indicate doubleRspo2and α-SMA labelling. Also observed are single-labeledRspo2mRNA+ cells found along the LP axis and in the subepithelial region (small arrow). Scale bar 100 μm. (d) Comparative localization ofRspo2mRNA and Gr1 in the colon of susceptible C3Ou mice 7 days post infection, seen at various magnification levels under dark-field or bright-field illumination. Large arrows indicateRspo2-positive cells and thin arrows indicate Gr1-positive cells mostly in subepithelial regions, in the lamina muscularis mucosae and in the submucosae (thin arrows). Scale bar: 500 μm (top panels), 100 μm (bottom panels). Data are representative of three independent experiments. CL, crypts of Lieberkühn; SM, sub-mucosae; Mu, mucosae; LMM, lamina muscularis mucosae; LP, lamina propria; SEP, subepithelial region; Ep, epithelia. Figure 3: Cri1 controls C. rodentium -induced Rspo2 expression within the colonic lamina propria. ( a ) Emulsion autoradiography detection of Rspo2 mRNA antisense labelling (as) by in situ hybridization (ISH) or control (s) hybridization in the colon mucosa seen as bright under dark-field illumination in susceptible C3Ou or resistant C3Ou.B6-Cri1 at 6 days post infection. Signal was detected in the microscopical loci seen in the bottom (large arrow) and close to luminal pole (small arrow) of the lamina propria; the same sections with cresyl violet staining (right). Scale bar 200 μm. ( b ) Enlarged view of Rspo2 -positive cells in infected susceptible C3Ou mice, ISH labelling (arrow) is observed in the lamina propria, close to the colonic epithelia (top) and at the bottom of the gland (bottom). Scale bar 50 μm. ( c ) Comparative localization of Rspo2 mRNA and α-SMA in the colon of susceptible C3Ou mice 7 days post infection, seen at various magnification levels under dark-field (top left, top middle) or bright-field illumination (bottom left, bottom middle). Top right panel is an enlargement of the boxed area in the bottom middle panel. Bottom right panel is a control with sense labelling. Large arrowheads indicate double Rspo2 and α-SMA labelling. Also observed are single-labeled Rspo2 mRNA+ cells found along the LP axis and in the subepithelial region (small arrow). Scale bar 100 μm. ( d ) Comparative localization of Rspo2 mRNA and Gr1 in the colon of susceptible C3Ou mice 7 days post infection, seen at various magnification levels under dark-field or bright-field illumination. Large arrows indicate Rspo2 -positive cells and thin arrows indicate Gr1-positive cells mostly in subepithelial regions, in the lamina muscularis mucosae and in the submucosae (thin arrows). Scale bar: 500 μm (top panels), 100 μm (bottom panels). Data are representative of three independent experiments. CL, crypts of Lieberkühn; SM, sub-mucosae; Mu, mucosae; LMM, lamina muscularis mucosae; LP, lamina propria; SEP, subepithelial region; Ep, epithelia. Full size image Activation of Wnt signalling in the colon of susceptible mice Histological analysis of hematoxylin and eosin-stained FFPE sections showed a significant impact of the Cri1 locus on the kinetics of C. rodentium -induced epithelial hyperplasia ( Fig. 4a and Supplementary Fig. S5 ). At 3 and 6 days post infection, crypt lengths were significantly increased in C3Ou compared with C3Ou.B6- Cri1 mice ( Fig. 4a ). Using PCNA staining to monitor cellular proliferation, we also noted qualitative differences in epithelial proliferation ( Fig. 4b ). By day 6 post infection, proliferative cells were observed throughout the entire extent of the colonic epithelium in susceptible C3Ou mice with no non-proliferating differentiated compartment observable. In contrast, in resistant congenic mice, the boundary between the proliferative compartment and the differentiated epithelium was well maintained and proliferation was delayed ( Fig. 4b ). 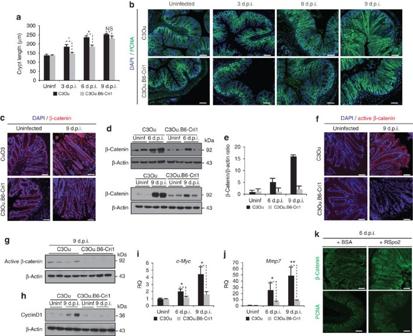Figure 4:Cri1controls crypt hyperplasia and canonical Wnt signalling activation duringC. rodentiuminfection. (a) Crypt length measurements in the distal colon of C3Ou (black bars) or C3Ou.B6-Cri1congenic mice (grey bars) left uninfected or at indicated time after infection (d.p.i., day post infection). (b) PCNA immunostained (green)/DAPI co-stained (blue) colon sections of C3Ou or C3Ou.B6-Cri1mice at indicated time points after infection (scale bar, 100 μm). (c) β-catenin immunostained (red)/DAPI co-stained (blue) colon sections of C3Ou or C3Ou.B6-Cri1mice left untreated or 9 days afterC. rodentiuminfection. Exposure times were the same for each sample and were optimized to avoid signal saturation in the C3Ou sample (scale bar, 50 μm). (d) Lysates of distal colon samples were assayed for β-catenin levels by immunoblotting. (e) Densitometry analysis of (d). (f–g) Immunodetection of dephosphorylated active β-catenin by immunofluorescence (f) or western blotting (g) in C3Ou or C3Ou.B6-Cri1mice (scale bar, 50 μm). Inf, exposure times were the same for each sample and were optimized to avoid signal saturation in the C3Ou sample. Immunoblot of CyclinD1 (h) and relative quantification by qPCR analysis ofc-MycandMmp7expression (i–j) in C3Ou or C3Ou.B6-Cri1mice (n>6). Data are representative of three independent experiments. (k) Recombinant R-spondin 2 (RSpo2) treatment induces epithelial proliferation and β-catenin activation. Representative images of β-catenin- (top) (scale bar, 50 μm) and PCNA- (bottom) (scale bar, 100 μm) stained colon sections of resistant C3Ou.B6-Cri1congenic mice, at 6 days after infection treated with recombinant RSpo2 or BSA. C3Ou.B6-Cri1were daily i.v. injected with hRSpo2 or equal amount of BSA from day 3 to day 5 after infection (day 3, 4: 50 μg; day5: 100 μg) (n=6). Data are representative of two independent experiments. Error bars in histograms represent s.e.m. *P<0.05; **P<0.01 (Mann-Whitney test) here and for all figures. Figure 4: Cri1 controls crypt hyperplasia and canonical Wnt signalling activation during C. rodentium infection. ( a ) Crypt length measurements in the distal colon of C3Ou (black bars) or C3Ou.B6- Cri1 congenic mice (grey bars) left uninfected or at indicated time after infection (d.p.i., day post infection). ( b ) PCNA immunostained (green)/DAPI co-stained (blue) colon sections of C3Ou or C3Ou.B6- Cri1 mice at indicated time points after infection (scale bar, 100 μm). ( c ) β-catenin immunostained (red)/DAPI co-stained (blue) colon sections of C3Ou or C3Ou.B6- Cri1 mice left untreated or 9 days after C. rodentium infection. Exposure times were the same for each sample and were optimized to avoid signal saturation in the C3Ou sample (scale bar, 50 μm). ( d ) Lysates of distal colon samples were assayed for β-catenin levels by immunoblotting. ( e ) Densitometry analysis of ( d ). ( f – g ) Immunodetection of dephosphorylated active β-catenin by immunofluorescence ( f ) or western blotting ( g ) in C3Ou or C3Ou.B6- Cri1 mice (scale bar, 50 μm). In f , exposure times were the same for each sample and were optimized to avoid signal saturation in the C3Ou sample. Immunoblot of CyclinD1 ( h ) and relative quantification by qPCR analysis of c-Myc and Mmp7 expression ( i – j ) in C3Ou or C3Ou.B6- Cri1 mice ( n >6). Data are representative of three independent experiments. ( k ) Recombinant R-spondin 2 (RSpo2) treatment induces epithelial proliferation and β-catenin activation. Representative images of β-catenin- (top) (scale bar, 50 μm) and PCNA- (bottom) (scale bar, 100 μm) stained colon sections of resistant C3Ou.B6- Cri1 congenic mice, at 6 days after infection treated with recombinant RSpo2 or BSA. C3Ou.B6- Cri1 were daily i.v. injected with hRSpo2 or equal amount of BSA from day 3 to day 5 after infection (day 3, 4: 50 μg; day5: 100 μg) ( n =6). Data are representative of two independent experiments. Error bars in histograms represent s.e.m. * P <0.05; ** P <0.01 (Mann-Whitney test) here and for all figures. Full size image Wnt signalling was strongly activated upon infection in susceptible mice but not in resistant mice. Although C3Ou and C3Ou.B6- Cri1 mice had similar levels and membranous localization of β-catenin before infection, C3Ou mice displayed a striking cytoplasmic accumulation of total and activated β-catenin during infection, which was not observed in C3Ou.B6- Cri1 mice ( Fig. 4c–g ). As further evidence of β-catenin activation, we found the Wnt target genes encoding c-Myc, cyclinD1 and the matrix metallopeptidase 7 to be specifically induced in susceptible animals ( Fig. 4h–j ). Treatment of resistant congenic mice during C. rodentium infection with recombinant R-Spondin 2 protein induced β-catenin activation and a proliferative response as compared with control infected and BSA-treated animals, and similar to what is observed in susceptible mice ( Fig. 4k ). Overall, these observations demonstrate that Cri1 -mediated susceptibility is associated with functional activation of Wnt signalling and a proliferative response, through Rspo2 induction in infected mice. Loss of intestinal differentiation in susceptible mice Wnt/β-catenin signalling has a key role in colon homoeostasis, allowing maintenance of pluripotent colonic crypt stem cells and the continuous generation of undifferentiated transient amplifying precursors, which differentiate as they migrate up the crypts. This gives rise to differentiated absorptive epithelial cells and goblet cells, which are continually sloughed off and replaced every 3–4 days in mice. Wnt signalling is normally restricted to the proliferative compartment that comprises the bottom third of the colonic crypts: as the cells reach the midcrypt region, Wnt signalling is downregulated to allow cell cycle arrest and differentiation [19] . Because strong Wnt signalling is known to inhibit colonic epithelial differentiation [19] , [20] , and because loss of function of colonic epithelium has been proposed as a mechanism for C. rodentium susceptibility [11] , [12] , we hypothesized that Rspo2 induction in susceptible mice would lead to critical perturbations in the differentiation of the large intestinal epithelium. Indeed, a pronounced loss of colonic goblet cells was observed in susceptible animals, as indicated by Alcian blue staining ( Fig. 5a ) and by qPCR analysis of markers of differentiated goblet cells ( Fig. 5b ). Although there was a loss of goblet cells observed in resistant mice, it was minor and delayed compared with what was seen in susceptible mice ( Fig. 5a ). The markers of terminally differentiated enterocytes Slc26a3 and Car4 were also found to be dramatically downregulated in susceptible mice ( Fig. 5c ). Slc26a3 (previously known as Dra : downregulated in adenocarcinomas) encodes the major colonic Cl − /HCO 3 − exchanger, which is exclusively expressed in differentiated enterocytes [10] , [21] , [22] , and together with carbonic anhydrase IV ( Car4 ) forms a functional unit for intestinal electroneutral absorption of chloride [23] . Importantly, downregulation of Car4 has been independently linked to lethality after C. rodentium infection [11] , [12] and to excessive Wnt signalling in colonic crypts [20] . Consistent with these works, we found a dramatic loss of Car4 expression at the mRNA and protein levels, and a 1,000-fold downregulation of Slc26a3 transcript in infected susceptible C3Ou mice. The resistant congenic mice C3Ou.B6- Cri1 maintained a significantly higher expression of Slc26a3 and Car4 than the parental C3Ou mice ( Fig. 5c ). Mutations in Slc26a3 in humans and mice cause congenital chloride-losing diarrhoea [24] , [25] , thus providing a link between the consequences of Rspo2 induction and diarrhoeal disease. 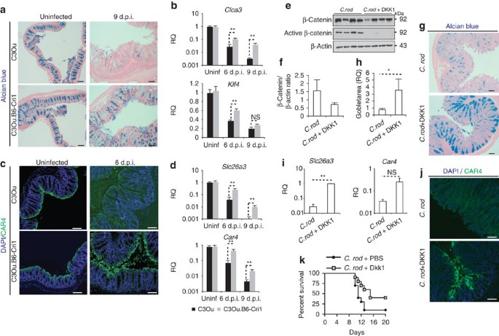Figure 5:Cri1controls loss of epithelial differentiation duringC. rodentiuminfection. Cri1controls level of goblet cell (a,b) and mature enterocyte (c,d) loss duringC. rodentiuminfection. (a) FFPE colon sections from C3Ou and C3Ou.B6-Cri1stained with Alcian blue (which stains mature goblet cells) ( × 20 magnification; scale bar, 100 μm). (b) qPCR analysis of the goblet cell markersClca3andKlf4in C3Ou versus C3Ou.B6-Cri1mice (n=6). (c) Immunodetection of CAR4 expression in enterocytes from C3Ou or C3Ou.B6-Cri1mice (scale bar, 100 μm). (d) qPCR analysis ofSlc26a3andCar4expression in C3Ou and C3Ou.B6-Cri1mice at various time points after infection (n=6). Data are representative of three independent experiments. (e–h) DKK1 treatment inhibits β-catenin activation and loss of epithelial differentiation duringC. rodentiuminfection. Susceptible C3Ou mice were infected withC. rodentiumand daily i.v. injected with recombinant DKK1 (C. rod+DKK1) or with PBS (C. rod) starting at day 3 post infection. (e) Lysates of distal colon samples were assayed for β-catenin levels by immunoblotting at day 7 post infection. (f) Densitometry analysis of (e). Alcian blue staining (g) and automatic quantification of level of intensity of Alcian blue staining (h) carried out with ImageJ software in sections of infected C3Ou mice, PBS or DKK1 treated at day 7 post infection (n=5) (scale bar, 100 μm). (i) Relative quantification by qPCR analysis ofSlc26a3andCar4expression and immunostaining of CAR4 (j) in DKK1-treated mice and PBS control mice at day 7 post infection (n=5) (scale bar, 100 μm). (k) Survival curve of C3Ou mice infected withC. rodentiumand treated with DKK1 or with PBS (n=10). Data are representative of two independent experiments. Error bars in histograms represent s.e.m. *P<0.05; **P<0.01 (Mann-Whitney test) here and for all figures. Figure 5: Cri1 controls loss of epithelial differentiation during C. rodentium infection . Cri1 controls level of goblet cell ( a , b ) and mature enterocyte ( c , d ) loss during C. rodentium infection. ( a ) FFPE colon sections from C3Ou and C3Ou.B6- Cri1 stained with Alcian blue (which stains mature goblet cells) ( × 20 magnification; scale bar, 100 μm). ( b ) qPCR analysis of the goblet cell markers Clca3 and Klf4 in C3Ou versus C3Ou.B6- Cri1 mice ( n =6). ( c ) Immunodetection of CAR4 expression in enterocytes from C3Ou or C3Ou.B6- Cri1 mice (scale bar, 100 μm). ( d ) qPCR analysis of Slc26a3 and Car4 expression in C3Ou and C3Ou.B6- Cri1 mice at various time points after infection ( n =6). Data are representative of three independent experiments. ( e – h ) DKK1 treatment inhibits β-catenin activation and loss of epithelial differentiation during C. rodentium infection. Susceptible C3Ou mice were infected with C. rodentium and daily i.v. injected with recombinant DKK1 ( C. rod +DKK1) or with PBS ( C. rod ) starting at day 3 post infection. ( e ) Lysates of distal colon samples were assayed for β-catenin levels by immunoblotting at day 7 post infection. ( f ) Densitometry analysis of ( e ). Alcian blue staining ( g ) and automatic quantification of level of intensity of Alcian blue staining ( h ) carried out with ImageJ software in sections of infected C3Ou mice, PBS or DKK1 treated at day 7 post infection ( n =5) (scale bar, 100 μm). ( i ) Relative quantification by qPCR analysis of Slc26a3 and Car4 expression and immunostaining of CAR4 ( j ) in DKK1-treated mice and PBS control mice at day 7 post infection ( n =5) (scale bar, 100 μm). ( k ) Survival curve of C3Ou mice infected with C. rodentium and treated with DKK1 or with PBS ( n =10). Data are representative of two independent experiments. Error bars in histograms represent s.e.m. * P <0.05; ** P <0.01 (Mann-Whitney test) here and for all figures. Full size image To demonstrate a direct link between activation of Wnt signalling and Cri1 -mediated susceptibility to infection, we treated infected susceptible mice with recombinant DKK1, a well-known antagonist of Wnt signalling. Notably, DKK1 treatment decreased C. rodentium -induced β-catenin accumulation and activation ( Fig. 5e ), increased levels of goblet cells ( Fig. 5g ) and increased Slc26a3 and Car4 expression ( Fig. 5i ) compared with mock-treated infected C3Ou mice. Daily DKK1 treatment of susceptible mice throughout the course of infection significantly increased survival compared with mock-treated infected mice (40% versus 10% survival; mean survival time 15 days versus 11 days; P -value <0.04) ( Fig. 5k ). Thus, inhibition of Wnt signalling through DKK1 administration counterbalances the C. rodentium -induced Wnt activation in susceptible mice leading to longer survival in treated animals. Mouse forward genetics is a powerful tool for the identification of genes and pathways important in biological process and has been very valuable for the characterization of key players in bacterial sensing, early response to infection and intestinal inflammation [26] , [27] . Here, we describe a single gene that naturally regulates susceptibility to enteric infection by C. rodentium in inbred mouse strains and uncover an unexpected link between bacterial sensing and intestinal homoeostasis. Our data lead us to propose a model where C. rodentium induces mucosal Rspo2 expression in susceptible mice, inducing proliferation of intestinal precursors and inhibiting differentiation of mature absorptive enterocytes and goblet cells, ultimately leading to the generation of a poorly differentiated epithelium and to fatal colitis ( Fig. 6 ). 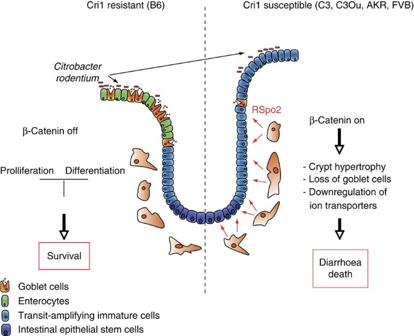Figure 6:A model for susceptibility toC. rodentiuminfection. Following infection,Rspo2is expressed in the colonic mucosa of susceptible mice. R-spondin 2 (RSpo2) triggers Wnt-pathway activation in transit-amplifying cells and leads to proliferation of immature precursors together with an inhibition in the differentiation of mature enterocytes and goblet cells. The resulting undifferentiated epithelium is no longer able to provide vital functions for fluid absorption, leading to lethal diarrhoea. Figure 6: A model for susceptibility to C. rodentium infection. Following infection, Rspo2 is expressed in the colonic mucosa of susceptible mice. R-spondin 2 (RSpo2) triggers Wnt-pathway activation in transit-amplifying cells and leads to proliferation of immature precursors together with an inhibition in the differentiation of mature enterocytes and goblet cells. The resulting undifferentiated epithelium is no longer able to provide vital functions for fluid absorption, leading to lethal diarrhoea. Full size image We previously measured colon weights in susceptible and resistant congenic mice on day 9 of C. rodentium infection and concluded that Cri1 did not impact intestinal hyperplasia at that time point [13] . However, the data we present here directly measuring crypt heights and cellular phenotypes throughout the course of infection demonstrate that intestinal proliferation following C. rodentium infection is, in fact, kinetically and qualitatively distinct in resistant and susceptible mice. Furthermore, we hypothesize that it is not hyperplasia per se , but rather, the loss of differentiated intestinal function that ultimately leads to death in susceptible strains. Genetic dissection of the Cri1 locus allowed us to define a critical interval, containing Rspo2 , that controls C. rodentium infection outcome. We also unambiguously associate mortality with upregulation of Rspo2 expression. However, the mechanisms that regulate Rspo2 expression in susceptible mice remain to be characterized. The minimal genetic interval for Cri1 contains a haplotype block specific to susceptible mouse strains and containing the proximal region of Rspo2 including the entire intergenic region between Eif3e and Rspo2 . We hypothesize that the genetic difference(s) underlying Rspo2 induction and susceptibility to infection localize to this region and confer differences in transcriptional regulation between resistant and susceptible mice. Identification of the specific genetic variations within this region that impact on Rspo2 transcriptional regulation is an important subject for further studies and will provide additional corroboration of the underlying mechanism of susceptibility in these mice. Tight regulation of the Wnt signalling pathway is critical to ensure normal function of the intestine, and maintaining a proper balance is key to intestinal health. Here we show that induction of robust Wnt signalling during intestinal infection is strongly correlated with mortality in susceptible mice. Conversely, stringent blockade of Wnt signalling through treatment of mice with a DKK1-expressing adenovirus markedly inhibited proliferation in the small intestine and colon, leading to progressive architectural degeneration, ulceration and death [28] . This suggests that the balance between too much and not enough Wnt signalling is a fine one, a concept that may be reflected in the relatively modest degree of rescue observed when we treated infected susceptible mice with recombinant DKK1. Constitutive activation of Wnt signalling constitutes the primary transforming event in colorectal cancer [29] . Recent findings have highlighted a critical role for the R-spondins in colonic carcinogenesis [18] , but to our knowledge a role for R-spondins in susceptibility to enteric infections has never been described. Our findings also provide a potential hypothesis for how the response to specific commensal or pathogenic bacteria may participate in the development of colorectal cancer. Furthermore, our own analysis of the data from the First International Inflammatory Bowel Disease Genetics Consortium meta-analyses [30] , [31] reveal strong associations of RSPO3 with both Crohn’s disease and ulcerative colitis ( Supplementary Table S1, S2 ), providing some evidence that R-spondins may have a broader role in linking infection or inflammation with intestinal homoeostasis. Mesenchymal–epithelial interactions orchestrate hedgehog (Hh), bone morphogenetic protein (Bmp), and Wnt signalling in the intestinal crypts and are critical for proper morphogenesis of intestinal architecture and for appropriate maintenance of the intestinal stem cell niche [32] . Mesenchymal cells of the intestinal lamina propria are also emerging as important players in immune function, and subepithelial myofibroblasts in particular are known to participate in innate [33] and adaptive immunity in the gut [34] . Here we describe a new cross talk between the mesenchyme and the closely opposed epithelial compartment, impacting host tolerance against enteric pathogens, through R-Spondin 2 signalling. Our work illustrates a novel pathological pathway leading to fatal diarrhoea and highlights a major role for intestinal mesenchyme in enteric infection outcome. Lastly, while A/E pathogens still represent a clinical challenge with few therapeutic options, our work suggests that targeting the R-Spondin/Wnt signalling pathway could represent a new approach to treat A/E pathogen-induced diarrhoea. Mice Breeding and experimental procedures were carried out in accordance with the Canadian Council on Animal Care and approved by our local ethical committee. C57BL/6J, C3H/HeOuJ, FVB/NJ and AKR/J mice were purchased from the Jackson Laboratory (Bar Harbor, ME, USA). All animals were maintained in a specific pathogen-free facility at McGill University. The congenic mice were produced according to standard procedures for introgression of C57BL/6J c15 allele onto the C3H/HeOuJ genome (C3Ou.B6- Cri1 ) or introgression of C3H/HeOuJ allele into C57BL/6J genome (B6.C3Ou- Cri1 ). Briefly, F1 mice were backcrossed to the parental strain. The resulting N2 mice with the desired segment of chr15 were selected by genotyping and used for subsequent backcrossing to the parental strain. Males and females (backcross generation N9) that inherited the intact derived congenic segment were intercrossed. Then, the offspring were genotyped to identify homozygotes for the desired segment, which were then intercrossed to maintain the line. To produce congenic sub-lines, F1 hybrids, made by crossing the congenic line to the recipient strain, were backcrossed to the recipient strain. Littermates issued from these backcrosses, characterized by recombination events within the Cri1 locus, were selected by genotyping polymorphic SNP markers. The selected recombinant mice were then backcrossed again to the recipient strain. Males and female mice issued from this backcross (heterozygous for the reduced introgressed region) were intercrossed to fix the recombinant chromosome in the homozygous state. The Cri1 homozygous offspring were selected for brother–sister mating and foundation of the new congenic sub-lines. Genotyping DNA was extracted from biopsies of mouse tails with overnight digestion in lysis buffer and proteinase K, followed by a chloroform extraction. The complete list of genetic markers used for genotyping of congenic lines is included in the Supplementary Methods. In-house PCRs done for mouse genotyping were sent to Genome Quebec (Montreal, QC, Canada) for sequencing. PCR was performed using standard touchdown PCR methods with primers obtained from the Mouse Genome Informatics website ( http://www.informatics.jax.org ). In vivo C. rodentium infection Five-week-old male or female mice were inoculated with C. rodentium strain DBS100. Bacteria were grown overnight in 3 ml of Luria-Bertani (LB) medium shaking at 37 °C. Mice were infected by oral gavage of 0.1 ml of LB medium containing 2–3 × 10 8 colony-forming units (CFUs) of C. rodentium . The infectious dose was verified by plating of serial dilutions. For survival analysis, animals were monitored daily and moribund animals were euthanized by CO 2 when clinical endpoints were achieved [13] . Animals were euthanized on experimental days 3, 6, 9 or 13 and their colons isolated and processed for histological examination and immunostaining or snap frozen for RNA/protein isolation. In some experiments, mice were daily intravenously injected with human recombinant R-spondin 2 protein (250 μg ml −1 in PBS, R&D systems) from day 3 to day 5 after infection. For treatment with recombinant DKK1, mice were injected with DKK1 (intravenous, 25 μg per day from day 3 to day 10 post infection and intraperitoneally 50 μg per day from day 11 to day 20). Production of recombinant DKK1 is described in Supplementary Methods . BM chimeras For BM chimera experiments, recipient mice were lethally irradiated (950 rad per 9.5 Gy) 24 h before reconstitution with BM from the indicated donor line. BM was aseptically harvested from tibia and femur of the respective donor strain, and 5–10 × 10 6 cells were injected into the tail vein of the irradiated recipients. Mice received antibiotics (Baytril) in the drinking water during the following 2 weeks after BM transfer and were allowed to reconstitute for a total of 8 weeks before being infected with C. rodentium . Chimerism ≥90% was validated by genotyping cell-sorted CD45+ splenocyte and tail DNA of chimeric mice with the polymorphic marker D15MIT229. Histopathology and immunofluorescence Distal colon sections were fixed in 10% buffered formalin, paraffin-embedded, sectioned at 5 μm, and subsequently stained with hematoxylin and eosin or Alcian blue using current procedures and visualized with a Zeiss axioscope microscope. Proliferative responses in infected tissues were scored in a blinded fashion by an expert veterinary pathologist. The average depth of 30 well-oriented colonic crypts was measured for each mouse. ImageJ software (Rasband, WS, ImageJ, http://rsb.info.nih.gov/ij ) was used to quantify differences in Alcian blue staining between samples. To standardize measurements, all images were taken immediately after staining using identical camera settings. Immunofluorescence was performed on paraffin sections. The slides were de-paraffinized with xylene twice for 5 min. The sections were rehydrated in ethanol 100% twice for 5 min, followed by 90%, 70% ethanol and water, 5 min each. The slides were then incubated for 10 min in boiling 0.1 M citrate buffer (pH 6.0) for antigen retrieval. PBS 0.2% Tween 20 was used as wash buffer. After blocking in PBS, 10% FCS and 1% BSA for 1 h at 37 °C, tissues were incubated with primary antibodies against PCNA (Abcam, cat. no. ab2426), β-catenin (BD, cat. no. 610154), active β-catenin (Millipore, cat. no. 05-665), CAR4 (R&D system, cat. no. AF2414), at a dilution of 1:100 in PBS 1% BSA for 1 h at 37 °C. This step was followed by a 1-h incubation with either Alexa-488-coupled goat anti-rabbit, Alexa-488-coupled goat anti mouse, Alexa-488-coupled donkey anti-goat, respectively. Tissues were counterstained with 1:100 4′,6-diamidino-2-phenylindole (DAPI) for DNA staining (Sigma) and mounted using ProLong Gold Antifade reagent (Invitrogen, Carlsbad, CA). Sections were viewed on a Zeiss AxioImager microscope and images were obtained using a Zeiss AxioCam HRn camera operating through AxioVision software. Quantitative real-time PCR Mice were euthanized at indicated time points by CO 2 asphyxiation. The penultimate centimetre of colon was dissected and immediately snap frozen in liquid nitrogen. Samples were then stored at −80 °C until processed. RNA from all tissue samples was isolated using Trizol reagent (Invitrogen) according to manufacturer’s directions. Samples were DNase treated using TURBO Dnase (Ambion). Complementary DNA was synthesized with SuperScript III Reverse Transcriptase (Invitrogen), using an Eppendorf PCR thermal cycler and random primers (Invitrogen). The purity of the samples was assessed spectrophotometrically; all samples had OD260/280 ratio between 1.8 and 2.0. Expression levels of the genes within Cri1 locus were assessed with TaqMan Gene Expression Assays (Applied Biosystems) on Applied Biosystems StepOne Plus Real-Time PCR system. For other genes, SYBR Green PCR reaction mix (10 μl) was composed of 5 μl of Light Cycler 480 SYBR Green I master (Roche), 4.5 μl of diluted cDNA and a final concentration of 1 μM of each primer. Sequences of primers are in the Supplementary Methods. Primers were designed with sequences spanning exon–exon junctions or with a separation of at least one intron on the corresponding genomic DNA. Correct efficiency of primers was controlled by PCR reactions performed on serial dilutions of cDNA. PCR reactions were done using a Light Cycler 480 system (Roche). Immunoblotting Colonic tissues samples were homogenized in B150 lysis buffer (20 mM Tris-HCl pH 8.0, 150 mM KCl, 10% glycerol, 5 mM MgCl 2 and 0.1% NP40) supplemented with Complete-mini protease inhibitor (Roche). Equal protein aliquots were subjected to SDS–PAGE (10% acrylamide) under reducing condition and proteins were transferred to a 0.2-mm PVDF membrane (Bio-Rad). Blots were blocked with 5% skimmed milk overnight at 4 °C, incubated with primary antibody against β-catenin (1:1000) (Cell Signaling, cat. no. 9562), active β-catenin (Millipore, cat. no. 05-665), CyclinD1 (Thermo Scientific, cat. no. RM 9104) or β-actin (1:10.000) (Sigma, cat. no. A 1978) for 1 h at room temperature. Detections were done with appropriate horseradish peroxidase-conjugated secondary antibody and a chemiluminescent substrate (Millipore). In situ hybridization ISH was performed using 35 S-UTP-labeled riboprobes synthesized in vitro from the Rspo2 DNA template (NM_172815.3) with forward T7 primer: 5′-GCGCTATAATACGACTCACTATAGGGAGATAGCTCAGGCAGCGAGAAACTTCA-3′ and reverse SP6: 5′-GCATTAATTTAGGTGACACTATAGAAGCGGCTGCAACCATTGTCCTTCGAACA-3′. RNA probes were synthesized in vitro from a DNA template of 950 nts, antisense and sense with SP6 and T7 RNA polymerase activities, respectively, and radiolabeled with 35 S-UTP (>1.000 Ci mmol −1 ; cat. no. NEG039H, PerkinElmer LAS Canada, Inc.). The 5 μm FFPE sections were treated with Proteinase K (0.1 mg ml −1 ) for 10–15 min. 35 S-labeled cRNA antisense and sense probes were used. Sections were hybridized overnight at 55 °C in 50% deionized formamide, 0.3 M NaCl, 20 mM Tris-HCl, pH 7.4, 5 mM EDTA, 10 nM NaPO 4 , 10% dextran sulphate, 1 × Denhardt’s, subjected to stringent washing at 65 °C in 50% formamide, 2 × SSC, and 10 mM DTT, followed by washing in PBS before treatment with 20 μg ml −1 RNAse A at 37 °C for 30 min. After washes in 2 × SSC and 0.1 × SSC for 10 min at 37 °C, the slides were dehydrated, opposed to an X-ray film for 5 days and then subjected to emulsion autoradiography. The autoradiography was revealed by treatment withD19 (Kodak) and sodium thiosulfate. We used frozen tissues cut into 6-μm sections for the combined ISH and immunocytochemistry (ICC). Tissues were divided into two groups: first group with ICC and second group without ICC. In addition to fixation in 4% formaldehyde, both groups were treated with triethanolamine/acetic anhydride, washed and dehydrated with ethanol series and then submitted to a classical procedure. For subsequent ICC, tissue was treated with 3% H 2 O 2 in water for 10 min to remove non-specific background, again washed with PBS and then pre-treated using heat-mediated antigen retrieval with sodium citrate buffer (pH=6) for 20 min. Primary antibodies anti Gr1 (Ebioscience, cat. no. 14-5931-81) and anti-α-SMA (Abcam, cat. no. ab5694) were diluted 1:100 in 1% BSA/PBS and incubated overnight at 4 °C. Immunoreaction was revealed using anti-rabbit- (or anti-rat) biotinylated second antibody (1:250) followed by HRP (Vector). The staining appears brown under light-field illumination. Tissue was then lightly stained with cresyl violet and mounted under cover slips. Statistics Statistic differences between pairs of survival curves of mice grouped by genotype were calculated using log-rank tests. Gene expression data were analysed by the Mann–Whitney test. * P <0.05; ** P <0.01; *** P <0.001 How to cite this article: Papapietro, O. et al . R-Spondin 2 signalling mediates susceptibility to fatal infectious diarrhoea. Nat. Commun. 4:1898 doi: 10.1038/ncomms2816 (2013).